A Bayesian modelling framework for tornado occurrences in North America Tornadoes represent one of nature’s most hazardous phenomena that have been responsible for significant destruction and devastating fatalities. Here we present a Bayesian modelling approach for elucidating the spatiotemporal patterns of tornado activity in North America. Our analysis shows a significant increase in the Canadian Prairies and the Northern Great Plains during the summer, indicating a clear transition of tornado activity from the United States to Canada. The linkage between monthly-averaged atmospheric variables and likelihood of tornado events is characterized by distinct seasonality; the convective available potential energy is the predominant factor in the summer; vertical wind shear appears to have a strong signature primarily in the winter and secondarily in the summer; and storm relative environmental helicity is most influential in the spring. The present probabilistic mapping can be used to draw inference on the likelihood of tornado occurrence in any location in North America within a selected time period of the year. Tornadoes represent one of nature’s most hazardous phenomena, capable of causing significant destructions and devastating injuries and fatalities. In May of 2011, the single deadliest tornado event in history occurred with 158 deaths in Joplin, Missouri [1] . Over the same year, tornadoes in the United States caused a total of over $28 billion in property damages [1] . Canada has also experienced significant losses caused by tornado activity, with significant tornado events occurring in recent years (for example, 14 tornadoes on 2 August 2006; 18 tornadoes on 20 August 2009) [2] . These events have brought the study of tornado activity to the forefront of climatological research, raising questions regarding the relative influence of large-scale climatic signals and the importance of delineating the role of the underlying atmospheric processes at the appropriate spatiotemporal scale. Tornado climatology represents a significant source of information used by a wide variety of groups, such as weather forecasters and researchers, emergency managers, civil engineers and insurance companies alike. Generally, the probability of tornado occurrence is derived from gridded values of tornado observations coupled with smoothing methods (for example, kernel densities) that are typically applied to delineate large-scale spatial patterns and to subsequently improve estimates for any single location [3] , [4] . However, these approaches rarely associate large-scale tornado variability with atmospheric variables that vary on relevant climatic timescales [5] , [6] . Predicting tornado activity from surrogate variables of the associated atmospheric processes can overcome issues related to data quality, particularly in areas where tornado observations are unreliable to form the basis of robust inference, due to either population density biases and/or the rarity of occurrence [2] , [7] . More importantly, the explicit consideration of large-scale climatic processes can shed light on the principal mechanisms of tornadogenesis and assess tornado frequency under different climate change scenarios or climate analogue studies [6] . Characterization of the interplay between large-scale atmospheric processes and local conditions leading to tornado formation has been examined in the severe storm research community [7] , [8] , [9] . Atmospheric variables such as convective available potential energy and vertical wind shear have been shown to be most relevant to mechanisms related to severe thunderstorm and tornado formation [7] . Conditions conducive to more intense tornadoes (F2–F5) appear to be more distinguishable than lower-end tornadoes (F0–F1), particularly by vertical shear parameters [9] , [10] , [11] . It has also been recognized that favourable conditions for tornado formation tend to vary seasonally. Namely, cool-season tornadoes are predominantly related to high vertical wind shear/low buoyancy regimes, particularly for more intense (F2–F5) tornadoes, relative to the considerably greater buoyancy/high shear conditions generating tornadoes in the warm season [12] , [13] , [14] , [15] , [16] , [17] . Recent research has also shown that the convective storm morphology and near-storm environment associated with tornadoes have clear seasonal and geographic patterns [11] , [18] , [19] ; notably, spring tornadoes in the Great Plains are produced by discrete, supercellular storms as compared with the predominantly quasi-linear convective systems in the Ohio Valley and the southeast United States [11] , [18] , [20] . Evidence that the prevailing conditions conducive to tornado occurrence exhibit clear seasonal and geographical variability leads us to hypothesize that the detailed characterization of their spatiotemporal patterns may address the current predictive deficiencies and consequently advance our capacity to effectively develop prognostic tools for tornado occurrence. In this study, the main objective is to delineate the seasonal and geographic variability of the relationship between large-scale climatological/atmospheric variables and both F0–F5 and F2–F5 tornado occurrence. Our analysis identifies the optimal combination of atmospheric variables and explicitly considers the sampling biases in tornado observations to collectively predict the monthly and seasonal tornado activity in North America. Specifically, we use Bayesian inference techniques to dissect the problem of tornado occurrence into a two step-process, in which we first consider the causal linkages between atmospheric variables and tornado activity in space and time, and we then postulate that the likelihood to observe a tornado is closely related to the population density. A conditional autoregressive term is also introduced in the statistical formulation to explicitly accommodate the serial correlation patterns of model residuals. Our ultimate goal is to develop an empirical modelling tool that can be used for drawing inference on the frequency of tornado occurrence or exceedance of a threshold number of tornadoes in any location in North America within a selected time period of the year. 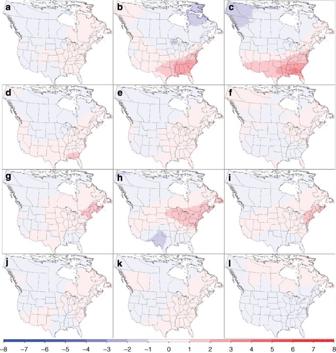Figure 1: Differences in the conditional autoregressive term between the CAPE–HLCY F0–F5 and CAPE–HLCY–VWSH F0–F5 monthly models. (a) December; (b) January; (c) February; (d) March; (e) April; (f) May; (g) June; (h) July; (i) August; (j) September; (k) October; (l) November. Model performance and posterior parameter patterns We investigated seven combinations of predictor variables to predict the tornado occurrence (F0–F5 and F2–F5) for each calendar month and season independently ( Supplementary Table 1 ). All of the predictor variables were standardized to examine their relative importance and possibly control any multicollinearity issues. We used two criteria to identify the optimal model configuration: (i) model performance as depicted by the deviance values or −2·log[model likelihood] ( Supplementary Tables 2 and 3 ) and (ii) the identifiability patterns of the parameter posteriors. When combined with CAPE, models with SHEAR and to a lesser extent with VWSH tended to perform better than the ones with HLCY in February to May. HLCY and SHEAR improved performance in June and July, respectively. VWSH tended to improve model performance in late summer-early autumn, while SHEAR outperformed the rest of the potential predictors throughout autumn until December. Interestingly, when reproducing F2–F5 tornadic activity, model performance with HLCY became better in January and VWSH improved model fit in June. On the basis of the two criteria of model performance and parameter identification, we inferred that the optimal model considers the variables CAPE, HLCY, VWSH to predict monthly values of F0–F5 and F2–F5 tornado counts. (Notably, the post hoc implementation of the deviance information criterion values suggests that the same model is not only the highest performing, but also the most parsimonious one in the majority of the cases examined.). The corresponding parameter posterior means and s.d. are shown in Tables 1 and 2 , respectively. Results for the rest of the models examined are shown in Supplementary Tables 4–15 . Table 1 Posterior parameter mean and s.d. values of the highest-performing model that considers the variables CAPE, HLCY and VWSH to predict F0–F5 tornadoes. 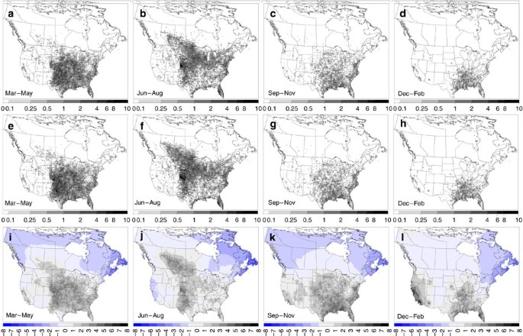Figure 2: Results of the CAPE–HLCY–VWSH F0–F5 model. The observed tornado counts per 100km2·yr−1,Tobs: (a) Spring; (b) Summer; (c) Autumn; (d) Winter; the predictions of the total number of tornado occurrence per 100km2·yr−1,Tlatent: (e) Spring; (f) Summer; (g) Autumn; (h) Winter; values for the conditional autoregressive term,ϕ: (i) Spring; (j) Summer; (k) Autumn; (l) Winter. Full size table Table 2 Posterior parameter mean and s.d. values of the highest-performing model that considers the variables CAPE, HLCY and VWSH to predict F2–F5 tornadoes. Full size table The posteriors of the standardized regression coefficients were characterized by clear seasonal patterns, which were consistent across all models tested. According to our modelling analysis, CAPE has a predominantly positive influence on tornado activity during the summer months (June to August) and a secondary (but distinct) one in February. VWSH demonstrated its strongest positive linkage with the tornado occurrence during winter months (December to March) and to a lesser extent in summer. The signature of HLCY was more distinct during the spring (March–April) and somewhat weaker in late fall and winter for the F0–F5 and F2–F5 models, respectively. Interestingly, although it was not included in the highest-performing model among the combinations examined, SHEAR was characterized by fairly similar seasonal patterns with VWSH with respect to its influence on model predictions (see Supplementary Tables 4–15 ). Regarding the relative importance of the different predictors, the standardized regression coefficients suggest that VWSH is most closely related to the variability of tornado occurrence (F0–F5 and F2–F5) in the winter, and together with CAPE appear to shape the tornadic activity in the summer. HLCY is more influential in early spring, although its posterior standardized mean values are slightly lower than those for VWSH (and SHEAR). Our analysis revealed several identifiability issues with interesting implications about the relative significance of the different predictor variables, when considered collectively as predictors in modelling frameworks of tornadic activity. For example, the signature of VWSH was significantly compromised after the addition of SHEAR with F2–F5 models in spring and fall months (see posteriors in Supplementary Tables 9 and 13 ). On the other hand, SHEAR is well identified with a distinct signature across all the F2–F5 models, with September being the only exception. The HLCY posteriors remain fairly similar with respect to their absolute magnitude and identifiability by the addition of VWSH ( Tables 1 and 2 versus Supplementary Tables 4 and 5 ), whereas the addition of SHEAR influences HLCY more significantly during the fall and winter ( Supplementary Tables 4 and 5 versus Supplementary Tables 10 and 11 ). The posteriors of CAPE are well identified for all F0–F5 models as well as for F2–F5 models during the summer maximal activity. The signature of CAPE remains fairly well delineated and practically unaltered by the different permutations of the other (wind shear-related) predictor variables. The differences of the random effect terms, ϕ , between the two-predictor CAPE–HLCY and the three-predictor CAPE–HLCY–VWSH F0–F5 (F2–F5) models for each month are shown in Fig. 1 ( Supplementary Fig. 2 ). Substantial differences are found in January and February (southeast United States) and from June to August (Eastern Atlantic Canada/United States to the Great Lakes), where the magnitude of the autoregressive term ϕ from the CAPE–HLCY–VWSH model is smaller. Interestingly, these are also the months when the impact of VWSH is more distinct, and thus its inclusion into the model allows us to effectively capture the variability of tornado occurrence in the winter and summer. On the other hand, the spatiotemporal patterns of the ϕ term with the two models are practically identical during the spring and autumn months. Figure 1: Differences in the conditional autoregressive term between the CAPE–HLCY F0–F5 and CAPE–HLCY–VWSH F0–F5 monthly models. ( a ) December; ( b ) January; ( c ) February; ( d ) March; ( e ) April; ( f ) May; ( g ) June; ( h ) July; ( i ) August; ( j ) September; ( k ) October; ( l ) November. Full size image Seasonal variability characterized the posterior values of the population effect parameter, β . The highest values were derived for the winter months and the lowest ones during the summer, that is, a higher population density is needed to observe tornadoes during the former rather than the latter months ( Tables 1 and 2 ). Substituting β back into equation (2) to identify the population thresholds where nearly all tornadoes can be observed ( p i ( β )≥0.995), the threshold levels ranged from 6.2 to 7.2 persons km −2 for F0–F5 tornadoes, which is consistent with the findings of other studies [2] , [21] , and 6.4 to 14.0 persons km −2 for F2–F5 tornadoes ( Supplementary Figs 3 and 4 ). These predicted patterns may be related to the seasonal variability in the day length, which in turn affects the ability to observe tornadoes [22] . Moreover, because of the higher proportion of nocturnal tornadoes occurring in the winter months (10% in July to 40% in February for F2–F5 tornadoes), the daylight effect on the ability of observing tornadoes may be compounded [22] . Regarding the higher population threshold range derived for the F2–F5 tornadoes, we believe that it likely reflects the fact that significant tornadoes tend to be reported in more populated areas comparing with F0–F5 events. The latter assertion reflects the ‘damage-related’ nature of the tornado intensity estimates in the F-scale rating. Tornadoes are more likely to have a high F-scale rating in populated areas, where there is more infrastructural capital in their path [23] . Assessment of tornado occurrence in North America The spatial distribution of the 30-year observations, T obs, along with the corresponding predictions, T latent, for F0–F5 (F2–F5) tornadoes are shown in Fig. 2a–d and Fig. 2e–h ( Fig. 3a–d and Fig. 3e–h ), respectively. Additional information related to the results of the CAPE-HLCY F0-F5 and F2-F5 models is provided in Supplementary Figs 5 and 6 . The spatial patterns for T obs and T latent are qualitative similar, indicative of the satisfactory model performance. In quantitative terms though, there are areas where the predicted tornado occurrences were considerably larger than the observed ones, primarily in the central to northern Plains and the Canadian prairies. 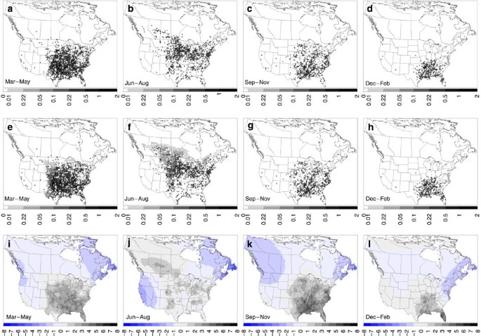Figure 3: Results of the CAPE–HLCY–VWSH F2–F5 model. The observed tornado counts per 100km2·yr−1,Tobs: (a) Spring; (b) Summer; (c) Autumn; (d) Winter; the predictions of the total number of tornado occurrence per 100km2·yr−1,Tlatent: (e) Spring; (f) Summer; (g) Autumn; (h) Winter; values for the conditional autoregressive term,ϕ: (i) Spring; (j) Summer; (k) Autumn; (l) Winter. The discrepancies were more pronounced during the spring and summer months ( Table 3 and Fig. 2e–h and Fig. 3e–h ; see also Supplementary Figs 8 and 9 for differences related to the CAPE-HLCY-VWSH model). Notably, the predominance of T latent i relative to T obs i is more evident in Canada than in the United States, suggesting a potentially significant sampling bias of tornado observations in the Canadian Prairies [2] ( Table 3 ). Figure 2: Results of the CAPE–HLCY–VWSH F0–F5 model. The observed tornado counts per 100km 2 ·yr −1 , T obs: ( a ) Spring; ( b ) Summer; ( c ) Autumn; ( d ) Winter; the predictions of the total number of tornado occurrence per 100km 2 ·yr −1 , T latent: ( e ) Spring; ( f ) Summer; ( g ) Autumn; ( h ) Winter; values for the conditional autoregressive term, ϕ : ( i ) Spring; ( j ) Summer; ( k ) Autumn; ( l ) Winter. Full size image Figure 3: Results of the CAPE–HLCY–VWSH F2–F5 model. The observed tornado counts per 100km 2 ·yr −1 , T obs: ( a ) Spring; ( b ) Summer; ( c ) Autumn; ( d ) Winter; the predictions of the total number of tornado occurrence per 100km 2 ·yr −1 , T latent: ( e ) Spring; ( f ) Summer; ( g ) Autumn; ( h ) Winter; values for the conditional autoregressive term, ϕ : ( i ) Spring; ( j ) Summer; ( k ) Autumn; ( l ) Winter. Full size image Table 3 Comparison between observed monthly numbers of tornadoes in Canada and the United States and those predicted by the CAPE–HLCY–VWSH model. Full size table In springtime, the global maximum for F0–F5 and F2–F5 tornado occurrences is located in the southern to central Plains, and extends eastward from Illinois to western Tennessee/Kentucky. F0–F5 T latent i predictions extend to southern Ontario and portions of Prairies in Canada but less so for F2–F5 tornadoes. Tornado occurrences in the summer shift northward to the central Plains and to the Prairies, and extends eastward to the Midwest, southern Ontario and the northeastern seaboard states. Note that there are peaks in eastern Colorado and Florida peninsula for F0–F5 tornadoes in the summer that are absent for F2–F5 tornadoes. These are predominately non-supercell tornadoes that are mostly of the lower F-scales [18] . It has been hypothesized from the tornado data that a sizable fraction of tornadoes across Canada are of the non-supercell type [24] . In the fall, areas of high tornadic activity shift south of the Prairies to the United States, east of the Rocky Mountains, characterized by a clear local minimum in the Appalachian Mountains. In the winter, the F0–F5 tornado maximum activity is located in the Gulf coast states, northward to Arkansas/Kentucky and in northern and central California coast. The random effects terms in the seasonal models demonstrate strong spatial covariance with the T latent posterior estimates in that the positive ϕ values typically coincide with higher T latent and vice versa ( Fig. 2i–l and Fig. 3i–l ). In other words, ϕ tends to compensate for the residual variability unaccounted for by the predictors included in the current model, although there were deviations from that pattern. For example, in the eastern United States and southern Ontario, where the tornado activity peaks up in the summer, ϕ i s are considerably lower than the Central United States (Colorado maximum) and Prairies. In the winter F0–F5 models, ϕ i s in the southwest United States have distinctly higher values than the southeastern region, despite the lower number of tornadoes in the west coast. While the likelihood of addressing the structural inadequacies of our model with the inclusion of additional predictors cannot be ruled out, we believe that an equally effective strategy may be to relax the assumption of common parameter values over the entire geographic domain. For modelling purposes, the delineation of regions that demonstrate greater homogeneity in their tornado activity and the subsequent configuration of a hierarchical structure, under which site-specific parameters will be used to describe the causal relationship between tornadic activity and atmospheric/climatological variables, may increase our capacity to accommodate the observed variability in space and time [2] . The expected tornado frequency, λ i , for the months when the highest F0–F5 and F2–F5 tornado occurrence is experienced in the United States (May) and Canada (July) are presented in Fig. 4 and Supplementary Fig. 7 for the CAPE-HLCY model. A wide area extending from Central United States to Illinois and onto western Tennessee in May is evident with high likelihood of F0–F5 tornadoes, resembling a clockwise rotated ‘C’ shape. For F2–F5 tornadoes, high likelihood rates are predicted in an extensive area around Oklahoma and Kansas. Relatively high F2–F5 tornado frequency rates are also predicted for Kentucky and (to a lesser extent) the Southern Great Lakes region. This pattern of tornadic activity shifts northward and extends east–west in July. Note that tornadoes predicted over the Great Lakes (that is, over water) are based on mechanisms related to tornado environments over land. They are not based on actual waterspout observations, but were included to give an indication of tornado occurrences and transition across the United States—Canada. 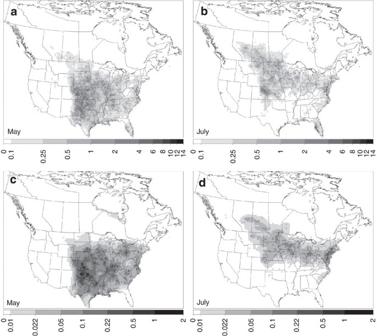Figure 4: Predictions of the CAPE–HLCY–VWSH model—Peak months of tornado activity for the United Stated and Canada. (a) May (F0–F5); (b) July (F0–F5); (c) May (F2–F5); (d) July (F2–F5) tornadoes. Figure 4: Predictions of the CAPE–HLCY–VWSH model—Peak months of tornado activity for the United Stated and Canada. ( a ) May (F0–F5); ( b ) July (F0–F5); ( c ) May (F2–F5); ( d ) July (F2–F5) tornadoes. Full size image North America experiences high tornado activity in the southern Great Plains and more broadly in the central United States during the springtime. According to our modelling analysis, CAPE, HLCY and VWSH (or SHEAR depending on the model examined) exert significant control and can offer a fairly accurate depiction of the spatial patterns. Tornado activity in the summer shifts north and Canada experiences its highest tornado occurrences in July. CAPE and VWSH are both important predictors in the summer. This finding reflects the transport of moisture from the Gulf of Mexico, occurrence of the elevated mixed layer [25] , and the poleward shift of jet stream, which in turn provide sufficient CAPE, large-scale upward motion and vertical wind shear to enhance majority of tornado activity. Non-supercell tornadoes are also common in the summer in Florida, eastern Colorado, northern Plains [18] and may represent a substantial fraction of the total number of occurrences in Canada [26] . Reflective of the latter assertion is the importance of CAPE (and weak HLCY and SHEAR signatures) in these regions, as updrafts (strong vertical shear) collocated along pre-existing vertical vortices enhance (prevent) non-supercell tornadoes [27] . During the fall season, the role of CAPE is minimized, while the influence of VWSH (and SHEAR) increases and the HLCY signature remains relatively constant. The mechanisms that generate tornadoes in the fall are more complicated and can be linked with different weather systems. In particular, tropical cyclones (TC) account for over 20% of all tornadoes in September (This number is based on the frequency of Gulf-landfalling TC-tornadoes from 1980 to 2008 (ref. 28 ) and the total number of tornado observations in this study). There are significant differences in the relative magnitudes of moisture, instability, shear and lift in conditions preceding TC tornadoes [29] . The smaller-scale boundaries associated with TC tornadoes are distinctly different from those of large-scale extratropical cyclones in spring and late autumn [30] . TC tornadoes are also associated with stronger lower troposheric vertical shear compared with those on the Great Plains [29] , which explains the stronger (weaker) and more (less) identifiable influence of SHEAR (VWSH), particularly for F2–F5 tornadoes. By contrast, almost all tornadoes in November stem from strong cold frontal systems, resembling to those in the spring season. Overall, this bimodal pattern may explain the change in the magnitude and/or sign of the standardized regression coefficients between September/October and November, reflecting a shift in the relative role of the different atmospheric variables. In winter, VWSH (and to a lesser extent SHEAR) is characterized by the highest-standardized slopes. This result is on parity with existing evidence from the literature that the influence of the subtropical jet to tornado activity is strongest in the winter, and can be a major factor of tornado formation and tornado outbreaks under extratropical storms [12] , [31] . Moreover, strong vertical wind shear (i) can play a role in organizing quasi-linear convective systems that can include individual or multiple supercells [32] and (ii) can produce a large vertical pressure gradient when horizontal vorticity is tilted and thus facilitates nocturnal convection to overcome large negative buoyancy, thereby producing tornadoes [33] . Thus, our finding that significant tornado occurrences in winter are closely associated with VWSH and SHEAR is a plausible result. The observations bias stemming from the differences in the population density was particularly evident in the Central/Northern Plains and the Prairies. Population thresholds for minimizing the likelihood of bias and observing all tornadoes ranged from 6 to 7.25 persons km −2 and 6 to 14 persons km −2 for F0–F5 and F2–F5 tornadoes, respectively. The higher values for F2–F5 may simply reflect the damage-based F-scale rating system, which could be biased towards populated area, where service- or infrastructure-related impacts can frequently be experienced [23] . The observation bias related to population density also appears to follow a seasonal pattern. Our modelling study suggests that highest population thresholds are needed to observe tornadoes during the winter months rather than the summertime. The different proportions of nocturnal tornadoes among the various periods of the year as well as the daylight variability may shape this pattern and determine the efficacy of the current monitoring systems. Overall, we showed that some of the spatial variability found in the actual tornado observations can be accounted for by the population density, and that our Bayesian modelling framework can effectively accommodate this observation bias. Model performance is better during the spring (winter) when HLCY (VWSH) is included, reflecting the seasonal variability of their causal association with tornado occurrence. Overall, the standardized regression coefficients had higher values with the F0–F5 than F2–F5 models, although substantial regional variability exists under the current model structure with seasonal or even monthly parameter specifications. The posterior estimates of the conditional autoregressive term delineated regional features that cannot be captured due to the structural inadequacy of a globally common parameterization and/or the absence of regionally relevant predictors/processes during different months of the year. Characteristic examples are the mid-level-specific humidity gradient, representing a measure of dry air intrusions which increases the propensity of tornadoes in TCs, may be important for tornado activity in August and September since a substantial number of tornadoes are related to landfalling TC from the Gulf of Mexico [28] or the strength of the low-level jet in the springtime, influencing the tornado activity in the South to Central Plains [34] . As recently shown [35] , there is a clear spatial distribution of the tornado environment that the current globally common parameter specification cannot address. This facet of our modelling framework will be investigated with a hierarchical model configuration in a subsequent study. In the context of tornado modelling, the adoption of a coarser temporal resolution (seasonal/monthly averages) is a significant distinction from the typically used predictor variables on shorter (subdaily) timescales [5] . This approach effectively postulates that atmospheric quantities varying on climate timescales can be used to draw inference about tornadic events with lifetime of no more than a few hours (and often only a few minutes) [5] , [6] . With this strategy, our intent is not to develop an early warning system, but rather to offer a modelling tool that can be used to characterize the frequency of tornado occurrence (or exceedance of a threshold number of tornadoes) in a particular location in North America within a selected period of the year, for example, probability of occurrence of more than one tornado in the selected four locations in May ( Fig. 5a,b ). In this regard, the present analysis resembles to modelling practices adopted in other disciplines (for example, aquatic ecology), where empirical models are in place to successfully reproduce the average prevailing conditions in a certain period of the year (summer growing season) and subsequently to predict the likelihood of occurrence of episodic events (end-of-summer hypoxia or cyanobacteria outbreaks) in a natural system. Thus, our modelling work is founded on the assumption that the association between average environmental conditions and ecological processes leading to short-term ecosystem shifts bears similarity to the connection between atmospheric quantities varying on climate timescales and tornado activity. The former linkage may be more evident as episodic ecosystem events are typically the escalation of a complex interplay among physical, chemical and biological processes that occur over a longer time period. In the context of tornadogenesis though, the time duration of the latter pattern with the atmospheric processes involved is distinctly shorter, and therefore the credibility of the present probabilistic mapping depends on the capacity of the changes in the moments (central tendency, spread) of the distribution of the environments occurring in the course of a month to faithfully capture the changes in the frequency of extreme subdaily environments (tails of the same distribution) associated with tornado occurrence. 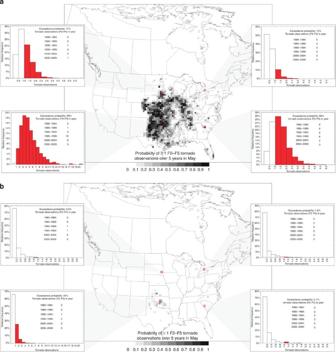Figure 5: Exceedance probability of one tornado event in May over the course of 5 years as predicted by the CAPE–HLCY–VWSH model. The four selected grid cells (indicated by the red boundaries) were Sioux Fall, South Dakota (Top left), Guelph-Waterloo, Ontario (Top right), El Reno, Oklahoma (Bottom left) and Edgefield county, South Carolina (Bottom right). The corresponding tornado events are also presented in 5-year time intervals during the study period 1980–2009. (a) F0–F5 tornadoes; (b) F2–F5 tornadoes. Figure 5: Exceedance probability of one tornado event in May over the course of 5 years as predicted by the CAPE–HLCY–VWSH model. The four selected grid cells (indicated by the red boundaries) were Sioux Fall, South Dakota (Top left), Guelph-Waterloo, Ontario (Top right), El Reno, Oklahoma (Bottom left) and Edgefield county, South Carolina (Bottom right). The corresponding tornado events are also presented in 5-year time intervals during the study period 1980–2009. ( a ) F0–F5 tornadoes; ( b ) F2–F5 tornadoes. Full size image Tornado counts and atmospheric data Canada tornado data covering the period 1980–2009 were collected from the updated national tornado database [2] , [24] , whereas the United States tornado data for the same period were collected from the Storm Prediction Center [36] . It is worth noting that the tornado data set used does not include tornadoes over water (that is, waterspouts) unless they made landfall; waterspout is a common occurrence over the Great Lakes in autumn. The annual number of tornadoes in Canada does not demonstrate any systematic long-term patterns, whereas the United States data suggest a slight increase in tornadic activity, stemming from an increase of F0 tornadoes ( Supplementary Fig. 1 ). There are no obvious trends for more intense tornadoes (F2–F5) in both countries. Although the temporal patterns of the total number of tornadoes over the 30-year study period are not substantially affected by non-meteorological factors, tornado reports are still hampered by sampling biases, mainly associated with population density, leading to underestimations in sparsely populated areas [23] , [37] , [38] . We computed a gridded climatology (30-year total) of monthly and seasonal tornado observations by counting the number of reported tornadoes for each calendar month and season via their tornado touchdown points in a geodesic 50 × 50 km grid ( Supplementary Data 1 ). This process was done separately for all tornadoes (F0–F5s) and for intense tornadoes (F2–F5s). The predicted spatial patterns of tornado occurrence, the population effects along with the corresponding population density thresholds are generally robust to the cell size of the grid configuration [2] . A range of atmospheric variables from 1980 to 2009 were obtained from the North American Regional Reanalysis [39] and their 30-year monthly and seasonally average values were calculated for consideration as potential predictors for our modelling framework ( Supplementary Table 22 ). North American Regional Reanalysis data were provided on a 32-km Lambert conformal grid, which were subsequently interpolated to match our grid. We selected the convective available potential energy (m 2 s −2 ) or CAPE as a measure of instability through the depth of troposphere that is related to updraft strength in thunderstorms. CAPE is widely used to quantify the subdaily atmospheric instability leading to tornado events [6] . Vertical wind shear is known to be very critical to tornadogenesis and different wind shear variables may be important in different types of tornado development. Thus, we explore the relative importance of three wind shear-related variables: (i) storm relative environmental helicity (m 2 s −2 ) or HLCY; a measure of the potential for cyclonic updraft rotation in right-moving supercells, it is calculated for the lowest 3 km layers above ground level [40] ; (ii) 0 to 6 km wind shear magnitude (m s −2 ) or SHEAR: a measure of wind shear from the surface through the mid-troposphere [41] . Strong vertical shear remove precipitation from updrafts, and induce vertical perturbation pressure gradients, so thunderstorms tend to become more organized and persistent; (iii) vertical wind shear from surface to tropopause (s −1 ) or VWSH: a measure of the upper-level wind speed normalized by the surface wind speed [42] . It is a measure of the upper-level jet strength inducing shear and vertical motion, and is often associated with severe weather. Strong upper-level jet streak tilts the storm as it rises vertically and has similar effects as SHEAR. Tornadoes can occur in a wide range of CAPE and wind shear levels that will be accommodated through systematic stratification by month/season and subsequent examination of the residual geographic variability. The considerable seasonality characterizing the actual values as well as the covariance patterns among CAPE and the three wind shear-related variables renders support to the latter strategy ( Supplementary Figs 10–12 ). Finally, since population-sampling bias creeps into tornado observations and may cause spurious geographical variability [23] , [37] , [38] , we adopted the Cheng et al .’s correction method [2] that uses population density data to quantify the observation error. Statistical framework For each month/season, we used a Bayesian modelling approach to decompose the problem of tornado occurrence into a series of conditional models coherently linked together via Bayes’ rule [2] , [43] . We specified a binomial model in which the observed (30-year) tornado counts in a particular month/season t for each grid cell i , T obs ti , are conditioned on the actual (but unobserved) tornado occurrences in the same month, T latent ti , and the probability of detection, p ti : The probability of detection p ti represents the likelihood to observe a tornado and is associated with the population density y i by the following exponential expression: where β t is the population effect parameter for month/season t and exp( y i ) is the exponential transformation of the original population density data in grid cell i . The actual occurrence of tornadoes, T latent ti , in the model domain is specified as a Poisson process, conditional on the average or expected tornado occurrence rate per grid cell λ ti , provided by the predictive model We use a log-linear model for λ ti given by the following expression: log( λ ti )= α t0 +α t1 x 1,ti +α t2 x 2,ti +...+ α tk x k,ti + ϕ ti , where x 1,ti , . . , x k.ti is a vector of the corresponding standardized monthly/seasonal atmospheric variables, α t0 is the model intercept, α t1 , . . , α tk are the regression coefficients and ϕ ti is a cell-specific random effect, capturing the residual variability of the tornado frequency in a particular month/season t and grid cell i , stemming from other explanatory factors/processes unaccounted for by the model. The inclusion of ϕ ti also aims to address the possibility that the signature of the regression coefficients may not be consistently strong in the tornado frequency records throughout the model domain [2] . It is also reasonable to assume that the random effects of the unaccounted factors have a regionalized/localized character and thus are spatially correlated. The characterization of the spatially correlated random terms ϕ ti was based on the Bayesian conditional autoregressive model [44] . The random error terms are jointly distributed as a multivariate normal distribution with mean 0 and an unknown covariance matrix. In particular, the model postulates that the spatial random effect in cell i depends on the neighbouring cells of i ( N i ) and that all of the neighbours have equal influence (weight of 1) on i . The term ϕ ti is defined by the conditional normal distribution ϕ ti ~ N ( μ ti , σ 2 / n i ), where and n i is the number of adjacent grid cells. Because we used a first-order neighbourhood approach and squared cells, N i represents the eight immediately adjacent cells. In this study, we opted for non-informative (or ‘flat’) prior distributions, reflecting no prior knowledge of the model parameters (see model codes in Supplementary Notes 1 and 2 ). A sequence of realizations from the model posterior were obtained using Markov chain Monte Carlo simulations. Convergence was assessed qualitatively by visually inspecting plots of the posterior Markov chains for mixing and stationarity and by inspecting density plots of the pooled posterior Markov chains for unimodality. We also assessed convergence quantitatively using the modified Gelman–Rubin convergence statistic [45] . The accuracy of the posterior parameter values was inspected by assuring that the Monte Carlo error for all parameters was less than 5% of the sample s.d. This process is undertaken independently for each month/season to assess the intra-annual variability of the models. We also conducted two additional exercises related to the predictive and structural confirmation of the present modelling framework ( Supplementary Figures 13–22 ). The first skill assessment test was based on splitting the 30-year data set into two subsets; namely, the calibration (1980–1994) and predictive validation (1995–2009) data sets. The former one was used to obtain parameter estimates through Bayesian updating and the derived model predictive posteriors were then tested independently against the latter ( Supplementary Table 23 ). The second skill assessment test aimed to examine the robustness of the inference drawn by the Binomial-Poisson model, given that the analysed tornado data have many zeros. The alternative statistical formulation was the zero-inflated Poisson model, based on a Zero-Inflated probability distribution that allows for frequent zero-valued observations. Structural confirmation of Bayesian modelling framework The second skill assessment test aimed to examine the robustness of the inference drawn by the binomial-Poisson model, given that the analysed tornado data have many zeros. The alternative statistical formulation was the zero-inflated Poisson (ZIP) model, based on a Zero-Inflated probability distribution that allows for frequent zero-valued observations [46] . This model is a statistical description of a random event, containing excess zero-count data per unit of time/space or within a fixed interval of a relevant covariate. The model dissects the studied event (tornado occurrence) into two components that correspond to two zero-generating processes. The first process reflects the sampling/observation error and is governed by a binary distribution that generates structural zeros, while the second mechanism represents the tornado occurrence rate and is governed by a Poisson distribution that generates counts, some of which may be zero. In the present model, the probability p of the former process is associated with the population density y and the mean λ of the latter process depends on the values of the causal factors (atmospheric predictors). The two model components can be described as follows: where T obs ti denotes the observed tornado counts in grid cell i and month/season t ; p ti represents the likelihood to observe a tornado in grid cell i and month/season t ; β t is the population effect parameter for month/season t ; exp( y i ) is the exponential transformation of the population density data in grid cell i ; λ ti is average or expected tornado occurrence rate per grid cell; x tij represents the standardized value of the j atmospheric variable in grid cell i and month/season t ; α t0 and α tj is the intercept and the j regression coefficients of the log-linear model used for λ ti , and ϕ ti is a cell-specific random effect, capturing the residual variability of the tornado frequency in a particular month/season t and grid cell i , stemming from other explanatory factors/processes unaccounted for by the model. Similar to the Binomial-Poisson model, we opted for non-informative (or ‘flat’) prior distributions, reflecting no prior knowledge of the model parameters (see Supplementary Notes 1 and 2 ). How to cite this article: Cheng, V. Y. S. et al . A Bayesian modelling framework for tornado occurrences in North America. Nat. Commun. 6:6599 doi: 10.1038/ncomms7599 (2015).